Targeting BIG3–PHB2 interaction to overcome tamoxifen resistance in breast cancer cells The acquisition of endocrine resistance is a common obstacle in endocrine therapy of patients with oestrogen receptor-α (ERα)-positive breast tumours. We previously demonstrated that the BIG3–PHB2 complex has a crucial role in the modulation of oestrogen/ERα signalling in breast cancer cells. Here we report a cell-permeable peptide inhibitor, called ERAP, that regulates multiple ERα-signalling pathways associated with tamoxifen resistance in breast cancer cells by inhibiting the interaction between BIG3 and PHB2. Intrinsic PHB2 released from BIG3 by ERAP directly binds to both nuclear- and membrane-associated ERα, which leads to the inhibition of multiple ERα-signalling pathways, including genomic and non-genomic ERα activation and ERα phosphorylation, and the growth of ERα-positive breast cancer cells both in vitro and in vivo . More importantly, ERAP treatment suppresses tamoxifen resistance and enhances tamoxifen responsiveness in ERα-positive breast cancer cells. These findings suggest inhibiting the interaction between BIG3 and PHB2 may be a new therapeutic strategy for the treatment of luminal-type breast cancer. Breast cancer is the most common cancer among women worldwide [1] , [2] . More than 70% of primary breast tumours are oestrogen receptor-α (ERα)-positive, and the interactions between oestrogen (E2) and ERα dramatically enhance the proliferative and metastatic activity of breast tumour cells [3] , [4] . E2 biological actions are mediated by both genomic and non-genomic mechanisms; in the former type nuclear ERα functions as a ligand-dependent transcription factor that regulates target gene expression levels [3] , [5] , whereas in the latter type E2-bound ERα in the plasma membrane associates with a variety of signalling molecules, including IGF receptor β (IGF-1Rβ), phosphoinositide 3-kinase (PI3K) and SH2 domain containing (Shc), which results in Akt and mitogen-activated protein kinase (MAPK) activation or increased nuclear ERα phosphorylation [6] , [7] , [8] , [9] , [10] . Thus, ERα has a pivotal role in the E2 signalling network and therefore represents an important therapeutic target for breast cancer. The selective ER modulator tamoxifen directly inhibits E2 and ERα interactions, and is a standard treatment offered to patients with ERα-positive breast cancer [11] , [12] , [13] . Nonetheless, tumours often develop resistance, leaving patients with recurrent tumours that lack targeted therapeutic options [14] , [15] . The potential mechanisms for either intrinsic or acquired endocrine resistance remain poorly understood, but they clearly include ERα-coregulatory proteins and cross-talk between the ERα pathway and other growth factors and kinase networks [10] , [11] , [16] . This knowledge has led to numerous treatment strategies combining endocrine and targeted inhibitor therapies [17] , [18] , [19] ; however, comprehensive measures for this problem remain unresolved. Therefore, identifying the factors and pathways responsible for resistance and defining ways to overcome it represent important therapeutic challenges in breast cancer research. The novel E2/ERα signalling regulator brefeldin A-inhibited guanine nucleotide-exchange protein 3 (BIG3), which is exclusively overexpressed in a majority of breast cancers, was recently identified from genome-wide expression profiles [20] , [21] . BIG3 interacts and colocalizes with prohibitin 2 (PHB2) in the cytoplasm of breast cancer cells [20] , [21] . PHB2 is known to function as a corepressor of ERα [22] , [23] . Our previous study demonstrated that when BIG3 was knocked down by small interfering RNA, E2 stimulation led to the nuclear translocation of a majority of the cytoplasmic PHB2, enhanced the interaction between PHB2 and ERα, and suppressed ERα transcriptional activity [21] . Accordingly, we hypothesized that BIG3 captures PHB2 in the cytoplasm of cancer cells and thereby inhibits the suppressive ability of PHB2 in the presence of E2, resulting in the constitutive activation of ERα signalling pathways. Here we describe a synthetic, cell-penetrating, dominant-negative peptide that inhibits the E2/ERα signalling network by activating the tumour suppressive ability of PHB2. This peptide also enhanced tamoxifen responsiveness and anti-tumour effects in tamoxifen-resistant (TAM-R) breast cancers. Thus, the regulation of E2 signalling by targeting the BIG3–PHB2 interaction introduces a new potential therapeutic approach for endocrine-resistant tumours, as well as ERα-positive breast cancers. Identification of the BIG3–PHB2 interacting region Previous studies have shown that the BIG3–PHB2 complex has a critical role in breast cancer cell growth [21] , and strategies capable of inhibiting this interaction may represent novel therapies for breast cancer. Therefore, we first attempted to determine the BIG3 region(s) required for the interaction with PHB2 through in silico and biochemical analyses. First, we independently cotransfected five partial constructs of FLAG-tagged BIG3 ( Fig. 1a ) with HA-tagged PHB2 (HA-PHB2) into COS-7 cells. Immunoprecipitation with an anti-FLAG antibody indicated that HA-PHB2 co-immunoprecipitated with BIG3 1–434 , BIG3 1–250 and full-length BIG3 ( Fig. 1b ), suggesting that the 101–250th amino acid region of BIG3 is minimally required for its interaction with PHB2. 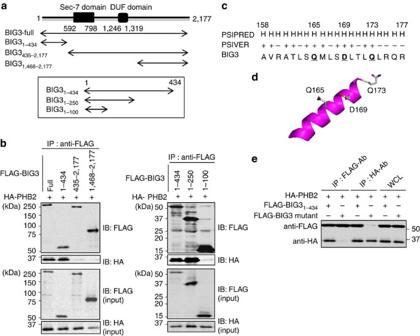Figure 1: Identification of the BIG3–PHB2 interacting region. (a) The schematic representation of human BIG3 and the five FLAG-BIG3 partial clones lacking one of the terminal regions is shown. (b) Immunoblot analyses were performed to identify the PHB2-binding region in BIG3. COS-7 cells were transfected with the indicated BIG3 constructs (full-length BIG3, BIG31–434, BIG3435–2,177, BIG31,468–2177, BIG31–100and BIG31–250) and HA-PHB2. After 48 h, the cells were lysed and FLAG-BIG3 was immunoprecipitated with an anti-FLAG antibody. Immunoprecipitated proteins and a portion of the original cell lysates (input) were immunoblotted as indicated. (c) The predicted interaction sites, as determined using PSIVER software, are shown. The underlined bold letters indicate the residues most likely to be involved in BIG3–PHB2 binding. (d) The putative PHB2-binding sites (Q165, D169 and Q173) on a predicted three-dimensional structure of BIG3 protein are shown. (e) Immunoblots were performed to assess the PHB2-binding region in BIG3 protein. The lysates from COS-7 cells transfected with BIG31–434or mutant BIG3 constructs were immunoprecipitated with anti-FLAG and anti-HA antibodies to detect BIG3 and PHB2, respectively. Full-length images of immunoblots are shown inSupplementary Fig. S9. Figure 1: Identification of the BIG3–PHB2 interacting region. ( a ) The schematic representation of human BIG3 and the five FLAG-BIG3 partial clones lacking one of the terminal regions is shown. ( b ) Immunoblot analyses were performed to identify the PHB2-binding region in BIG3. COS-7 cells were transfected with the indicated BIG3 constructs (full-length BIG3, BIG3 1–434 , BIG3 435–2,177 , BIG3 1,468–2177 , BIG3 1–100 and BIG3 1–250 ) and HA-PHB2. After 48 h, the cells were lysed and FLAG-BIG3 was immunoprecipitated with an anti-FLAG antibody. Immunoprecipitated proteins and a portion of the original cell lysates (input) were immunoblotted as indicated. ( c ) The predicted interaction sites, as determined using PSIVER software, are shown. The underlined bold letters indicate the residues most likely to be involved in BIG3–PHB2 binding. ( d ) The putative PHB2-binding sites (Q165, D169 and Q173) on a predicted three-dimensional structure of BIG3 protein are shown. ( e ) Immunoblots were performed to assess the PHB2-binding region in BIG3 protein. The lysates from COS-7 cells transfected with BIG3 1–434 or mutant BIG3 constructs were immunoprecipitated with anti-FLAG and anti-HA antibodies to detect BIG3 and PHB2, respectively. Full-length images of immunoblots are shown in Supplementary Fig. S9 . Full size image In parallel with this approach, we attempted to predict the protein binding sites on BIG3 using the PSIVER (Protein–protein interaction SItes prediction server) software [24] , and we identified a cluster of candidate binding residues within the 101–250th amino acid region. This cluster region contained three of the highest scoring (≥0.6) residues (Q165, D169 and Q173; Fig. 1c ), which were oriented in the same direction ( Fig. 1d ). Indeed, the BIG3 mutations in which all of these target residues were substituted with alanine almost completely abolished the interaction with HA-PHB2 ( Fig. 1e ), indicating the importance of Q165, D169 and Q173 for BIG3 heterodimerization with PHB2. Moreover, D169 was the most critical site among these residues for binding, although an alanine mutation on each residue resulted in reduced binding ( Supplementary Fig. S1 ). Accordingly, we focused on these residues as candidate PHB2-binding residues. A peptide with dominant-negative influence on ERα activity We next investigated the possibility of a cell-penetrating peptide as a dominant-negative inhibitor targeting the BIG3–PHB2 interaction, and designed a specific peptide that included these PHB2-binding residues to target the BIG3–PHB2 interaction. This peptide, referred to as ERα activity-regulator synthetic peptide (ERAP), contained the BIG3 potential binding residues (165– Q MLS D LTL Q LRQR–177) and membrane-permeable polyarginine residues (11R) at its NH 2 terminus ( Fig. 2a ). As negative controls, peptides containing a scrambled amino acid sequence (scrERAP) and either alanine mutations at key residues (mtERAP) were constructed ( Fig. 2a ). Indeed, co-immunoprecipitation experiments revealed that ERAP, but not mtERAP or scrERAP, completely inhibited the complex formation of endogenous BIG3 and PHB2 in the ERα-positive breast cancer cell lines MCF-7 and KPL-3C, which strongly express BIG3 and PHB2 ( Fig. 2b and Supplementary Fig. S2 ). We also examined the direct inhibition of the BIG3–PHB2 interaction using ERAP. As expected, HA-ERAP bound to His-tagged recombinant PHB2 protein and inhibited the BIG3–PHB2 interaction in a dose-dependent manner, whereas scrERAP did not ( Fig. 2c ). In addition, mtERAP exhibited modest binding to the PHB2 protein at levels substantially lower than ERAP ( Fig. 2c ). Surface plasmon resonance (BIAcore) interaction analysis revealed that ERAP bound to the His-tagged recombinant PHB2 with a dissociation constant (Kd)=18.9 μM ( Fig. 2d ). Thus, our data suggested that ERAP directly bound to PHB2, resulting in the specific inhibition of BIG3–PHB2 complex formation. 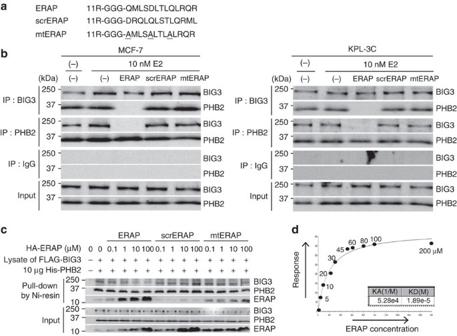Figure 2: ERAP inhibits the interaction of BIG3 with PHB2. (a) The ERAP, scrERAP and mtERAP sequences are shown. (b) The inhibitory effects of ERAP treatment on BIG3–PHB2 interactions were evaluated in MCF-7 (left) and KPL-3C cells (right). (c) Direct inhibition of the BIG3–PHB2 interaction by ERAP was evaluated. The lysates of COS-7 cells, transiently transfected with FLAG-BIG3, were incubated with 6 × His-tagged recombinant PHB2 (His-PHB2) and HA-ERAP, HA-scrERAP or HA-mtERAP for 1 h. Then, His-PHB2 was captured with Ni-NTA agarose, and the bound fractions were immunoblotted as indicated. (d)In vitrodirect interaction of ERAP and PHB2 was evaluated by BIAcore. Figure 2: ERAP inhibits the interaction of BIG3 with PHB2. ( a ) The ERAP, scrERAP and mtERAP sequences are shown. ( b ) The inhibitory effects of ERAP treatment on BIG3–PHB2 interactions were evaluated in MCF-7 (left) and KPL-3C cells (right). ( c ) Direct inhibition of the BIG3–PHB2 interaction by ERAP was evaluated. The lysates of COS-7 cells, transiently transfected with FLAG-BIG3, were incubated with 6 × His-tagged recombinant PHB2 (His-PHB2) and HA-ERAP, HA-scrERAP or HA-mtERAP for 1 h. Then, His-PHB2 was captured with Ni-NTA agarose, and the bound fractions were immunoblotted as indicated. ( d ) In vitro direct interaction of ERAP and PHB2 was evaluated by BIAcore. Full size image ERAP translocates PHB2 and attenuates nuclear ERα activation We investigated the subcellular distribution of endogenous PHB2 in breast cancer cells following ERAP treatment by immunocytochemical and biochemical approaches. In the presence of E2, treatment with ERAP, but not with scrERAP, led to a significant increase in the amount of nuclear PHB2 in a time-dependent fashion ( Fig. 3a ). In addition, in the presence of E2, ERAP treatment led to a decrease in cytoplasmic PHB2, thereby substantially increasing the interaction between PHB2 and ERα in the nucleus even after 1 h ( Fig. 3b ). Furthermore, ERAP co-immunoprecipitated and colocalized with endogenous PHB2 in the nucleus and the cytoplasm ( Supplementary Fig. S3a,b ) but did not directly bind to ERα or BIG3. These findings suggested that ERAP caused PHB2 to be released from BIG3 and led to E2-dependent PHB2 nuclear translocation, eventually resulting in the interaction of PHB2 with nuclear ERα in cancer cells. 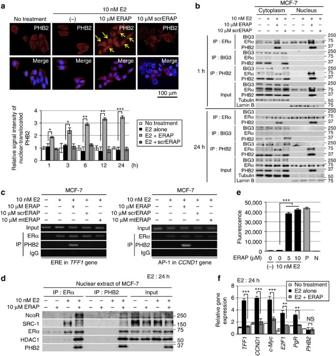Figure 3: ERAP promotes PHB2 nuclear translocation and suppresses E2-induced gene expression. (a) Upper, representative immunofluorescence images of the subcellular localization of PHB2 are shown; PHB2 (red), 4',6-diamidino-2-phenylindole (blue). The arrows indicate PHB2 nuclear translocation. Lower, statistical analyses of the nuclear intensity of translocated PHB2. The data are expressed as the fold increase over untreated cells set at 1.0 and represent the mean±s.e.m. of four independent experiments (*P<0.05, **P<0.01, ***P<0.001 in two-sided Student’st-test). (b) Immunoblot analysis was performed to detect the subcellular localization of ERα, BIG3 and PHB2 after immunoprecipitation with the antibodies against the indicated proteins in the presence of E2 and ERAP or scrERAP. α/β-Tubulin (tubulin) and laminin B were used as loading controls for the cytoplasmic and nuclear fractions, respectively. (c) ChIP assays were used to determine the recruitment of ERα and PHB2 to theTFF1ERE sequence (left) and theCCND1AP-1 motif (right) after 24 h of treatment. (d) Exchange of chromatin-remodelling complexes by ERAP. After treatment of MCF-7 cells for 24 h with E2±ERAP, the nuclear fractions were immunoprecipitated with anti-ERα or -PHB2 antibodies and were immunoblotted with antibodies against the indicated proteins. (e) Deacetylation of chromatin-remodelling complexes was evaluated after ERAP treatment. Nuclear extracts from HeLa cells and PBS were used as positive (P) and negative (N) controls, respectively. The data represent the mean±s.e.m. of three independent experiments (***P<0.001 in two-sided Student’st-test). (f) The effects of ERAP on ERα-target gene expression levels were evaluated using real-time PCR. The data are expressed the fold increase over untreated cells at 0 h (set at 1.0) and represent the mean±s.e.m. of three independent experiments (**P<0.01, ***P<0.001, NS, no significance in two-sided Student’st-test). Figure 3: ERAP promotes PHB2 nuclear translocation and suppresses E2-induced gene expression. ( a ) Upper, representative immunofluorescence images of the subcellular localization of PHB2 are shown; PHB2 (red), 4',6-diamidino-2-phenylindole (blue). The arrows indicate PHB2 nuclear translocation. Lower, statistical analyses of the nuclear intensity of translocated PHB2. The data are expressed as the fold increase over untreated cells set at 1.0 and represent the mean±s.e.m. of four independent experiments (* P <0.05, ** P <0.01, *** P <0.001 in two-sided Student’s t -test). ( b ) Immunoblot analysis was performed to detect the subcellular localization of ERα, BIG3 and PHB2 after immunoprecipitation with the antibodies against the indicated proteins in the presence of E2 and ERAP or scrERAP. α/β-Tubulin (tubulin) and laminin B were used as loading controls for the cytoplasmic and nuclear fractions, respectively. ( c ) ChIP assays were used to determine the recruitment of ERα and PHB2 to the TFF1 ERE sequence (left) and the CCND1 AP-1 motif (right) after 24 h of treatment. ( d ) Exchange of chromatin-remodelling complexes by ERAP. After treatment of MCF-7 cells for 24 h with E2±ERAP, the nuclear fractions were immunoprecipitated with anti-ERα or -PHB2 antibodies and were immunoblotted with antibodies against the indicated proteins. ( e ) Deacetylation of chromatin-remodelling complexes was evaluated after ERAP treatment. Nuclear extracts from HeLa cells and PBS were used as positive (P) and negative (N) controls, respectively. The data represent the mean±s.e.m. of three independent experiments (*** P <0.001 in two-sided Student’s t -test). ( f ) The effects of ERAP on ERα-target gene expression levels were evaluated using real-time PCR. The data are expressed the fold increase over untreated cells at 0 h (set at 1.0) and represent the mean±s.e.m. of three independent experiments (** P <0.01, *** P <0.001, NS, no significance in two-sided Student’s t -test). Full size image ERα has been shown to modulate transcription in two ways: (i) through direct binding to oestrogen-responsive elements (EREs) located in the promoter and/or enhancer regions of target genes [25] and (ii) by serving as a co-activator of other transcription factors such as AP-1 (ref. 26 ). Therefore, we explored the impact of ERAP treatment on these two modes of ERα transcriptional activity. First, we performed a chromatin immunoprecipitation (ChIP) assay with E2-stimulated MCF-7 cells. The results showed that ERAP treatment induced E2-dependent recruitment of the endogenous ERα–PHB2 complex on the ERα target genes, TFF1 and CCND1 , respectively, ( Fig. 3c ), suggesting that ERAP did not inhibit the ability of ERα to bind ERE or AP-1. In luciferase assays with ERE or AP-1 reporters, ERAP significantly inhibited both forms of E2-induced ERα transcriptional activity in a dose-dependent manner in MCF-7 and KPL-3C cells ( Supplementary Fig. S3c ), but no significant inhibition was observed with scrERAP or mtERAP. These results indicated that ERAP suppressed ERα transcriptional activity levels through both canonical ERE- and non-canonical AP-1-binding mechanisms. PHB2 is known to act as an ERα transcriptional corepressor by competing with the co-activator SRC-1 to bind ERα [23] and by recruiting histone deacetylase 1 (HDAC1; ref. 27 ) and another corepressor, NcoR [28] . Thus, we next explored the effect of ERAP on this recruitment in MCF-7 and KPL-3C cells using ChIP assays. Stimulation with E2 alone recruited SRC-1 to ERα, whereas ERAP treatment led to the direct association of PHB2 with ERα in the presence of E2, reduced SRC-1 binding to ERα, and enhanced the recruitment of HDAC1 and NcoR in MCF-7 ( Fig. 3d ) and KPL-3C cells ( Supplementary Fig. S3d ). Moreover, we performed a ChIP–quantitative PCR assay, with E2-stimulated MCF-7 cells. The results showed that ERAP treatment significantly reduced the E2-dependent recruitment of endogenous SRC-1 on the TFF1 gene but increased the E2-dependent recruitment of endogenous NcoR, HDAC1 and PHB2 ( Supplementary Fig. S3e ). In contrast, ERAP treatment had no effect on ChIP assay using an anti-BIG3 antibody ( Supplementary Fig. S3e ) or on ERα expression at the mRNA or protein level ( Supplementary Fig. S3f ). Subsequently, we investigated the HDAC activity of PHB2 immunoprecipitates in MCF-7 cells and found that the chromatin-remodelling complexes recruited by ERAP treatment led to a significant increase in HDAC activity ( Fig. 3e ). Moreover, ERAP significantly suppressed E2-induced expression of TFF1 , CCND1 , c-Myc , E2F1 and PgR [29] , [30] , [31] , [32] , [33] ( Fig. 3f ). In addition, we validated the suppressive effect of BIG3 on ERα transcriptional activity. BIG3 depletion caused a significant reduction in the canonical ERE and non-canonical AP-1 ERα transcriptional activities in ERα-positive MCF-7 cells but did not affect ERα-negative MDA-MB-231 cells ( Supplementary Fig. S3g ). Taken together, these findings indicated that nuclear-translocated PHB2 following ERAP treatment directly bound to ERα and acted as a corepressor by recruiting HDAC1 and NcoR, thereby leading to an almost complete suppression of the ERα target gene expression. ERAP suppresses E2-dependent non-genomic ERα signalling In addition to ERα acting as a nuclear transcription factor, E2 rapidly induces IGF-1Rβ tyrosine phosphorylation followed by the formation of a ternary complex of IGF-1Rβ, ERα and Shc in the cell membrane [9] , even though the abundance of membrane-bound and cytoplasmic ERα is low in primary breast cancers [34] . Indeed, we observed that a portion of PHB2 released from BIG3 by ERAP interacted with ERα in the cytoplasmic/plasma membrane cell fraction, regardless of the presence of E2 ( Fig. 3a,b and Supplementary Fig. S3a,b ). Therefore, we hypothesized that ERAP could also affect these non-genomic actions of ERα. First, we detected E2-induced tyrosine phosphorylation of IGF-1Rβ and co-immunoprecipitated IGF-1Rβ, ERα and Shc in both MCF-7 and KLP-3C cells ( Fig. 4a ), which highly expressed IGF-1Rβ and PI3K ( Supplementary Fig. S4a ), as described previously [9] . In contrast, ERAP treatment removed Shc from this complex and formed a new ternary complex consisting of IGF-1Rβ, ERα and PHB2, and thereby suppressed E2-induced tyrosine phosphorylation of IGF-1Rβ ( Fig. 4a ). We then examined the effects of ERAP on the phosphorylation of membrane-associated ERα (S118), because its phosphorylation has been associated with invasive breast cancer in clinical specimens [35] . ERAP treatment clearly suppressed the E2-induced phosphorylation (S118) of membrane-associated ERα in the IGF-1Rβ-precipitated membrane fraction of MCF-7 cells ( Supplementary Fig. S4b ). Moreover, ERAP also interfered with the E2-induced interactions of ERα and PI3K in both MCF-7 and KLP-3C cells ( Fig. 4b ). Next, we examined the effects of ERAP on the phosphorylation status of Akt and p42/44 MAPK, which are the downstream signalling molecules of IGF-1Rβ and PI3K, respectively. As expected, we observed that Akt (S473) and p42/44 MAPK (T202/Y204) phosphorylation levels were clearly increased in a time-dependent manner after E2 stimulation in both cell lines, whereas treatment with ERAP, but not scrERAP, completely suppressed the E2-induced phosphorylation levels of both proteins ( Fig. 4c and Supplementary Fig. S4c ). However, the PHB2 released from BIG3 following ERAP treatment did not directly interact with Akt or p42/44 MAPK ( Supplementary Fig. S4d ). Taken together, these results strongly suggested that ERAP interfered with E2-induced non-genomic ERα activation pathways, such as those mediated by IGF-1Rβ. 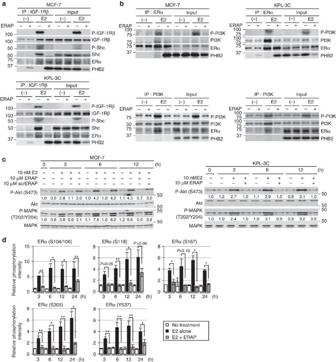Figure 4: ERAP regulates the E2-induced non-genomic pathway via IGF-1Rβ. (a,b) The inhibitory effects of ERAP on the interactions of ERα with IGF-1Rβ and Shc (a), and the interaction of ERα and PI3K (b) in MCF-7 and KPL-3C cells. (c) Immunoblot analyses were performed to evaluate the inhibitory effects of ERAP on E2-induced Akt (S473) and p42/44 MAPK (T202/Y204) activities in MCF-7 (left) and KPL-3C (right) cells. Representative results are shown from one of four independent experiments. (d) The inhibitory effects of ERAP were evaluated on E2-induced phosphorylation of ERα (S104/S106, S118, S167, S305 and Y537) in MCF-7 cells. The data are expressed as the fold increase over untreated cells at 0 h and represent the mean±s.e.m. of three independent experiments (*P<0.05, **P<0.01 in two-sided Student’st-test). Figure 4: ERAP regulates the E2-induced non-genomic pathway via IGF-1Rβ. ( a , b ) The inhibitory effects of ERAP on the interactions of ERα with IGF-1Rβ and Shc ( a ), and the interaction of ERα and PI3K ( b ) in MCF-7 and KPL-3C cells. ( c ) Immunoblot analyses were performed to evaluate the inhibitory effects of ERAP on E2-induced Akt (S473) and p42/44 MAPK (T202/Y204) activities in MCF-7 (left) and KPL-3C (right) cells. Representative results are shown from one of four independent experiments. ( d ) The inhibitory effects of ERAP were evaluated on E2-induced phosphorylation of ERα (S104/S106, S118, S167, S305 and Y537) in MCF-7 cells. The data are expressed as the fold increase over untreated cells at 0 h and represent the mean±s.e.m. of three independent experiments (* P <0.05, ** P <0.01 in two-sided Student’s t -test). Full size image ERAP represses E2-dependent ERα phosphorylation Accumulating evidence suggests that phosphorylation of ERα is an important regulator of E2-induced ERα transcriptional activity, DNA-binding, co-activator binding, and protein stability and cell proliferation in ERα-positive breast cancer cells [36] , [37] , [38] , [39] , [40] , [41] , [42] , [43] . Thus, we examined the effects of ERAP on ERα phosphorylation at sites, including S104/S106, S118, S167, S305 and Y537. Phosphorylation at these five sites within ERα was clearly increased in response to E2 stimulation and continued for at least 24 h in MCF-7 and KPL-3C cells. In contrast, treatment with ERAP completely abrogated these responses in both cell lines ( Fig. 4d and Supplementary Fig. S4e ). Collectively, these results clearly showed that PHB2 released from BIG3 following ERAP treatment reduced E2-dependent ERα phosphorylation, leading to ERα inactivation. ERAP suppresses E2-dependent breast cancer cell growth We elucidated the inhibitory effect of ERAP on the E2-dependent growth of MCF-7 or KPL-3C cells. Treatment with ERAP, but not scrERAP or mtERAP, significantly reduced E2-stimulated cell growth in a dose-dependent manner (IC 50 =2.2 μM and 1.9 μM in MCF-7 and KPL-3C cells, respectively; Fig. 5a ). Notably, ERAP doses greater than 5 μM completely abolished the proliferative response for up to 3 h after E2 stimulation ( Supplementary Fig. S5a ). The inhibition of both cell growth ( Supplementary Fig. S5b , left panel) and ERα transcriptional activity ( Supplementary Fig. S5b , right panel) was maintained for 24 h after ERAP treatment. We confirmed similar growth inhibitory effects of ERAP in other breast cancer cell lines expressing ERα, BIG3 and PHB2 (that is, ZR-75-1, HCC1500, BT-474, YMB-1, T47D, KPL-1 and HBC4; Supplementary Fig. S5c ). In contrast, ERAP had no effect on the growth of normal mammary epithelial MCF-10 A cells ( Fig. 5b ) that did not express ERα or BIG3 ( Supplementary Fig. S2 ). These findings suggested that ERAP specifically inhibited the growth of breast cancer cells without affecting normal mammary cells. 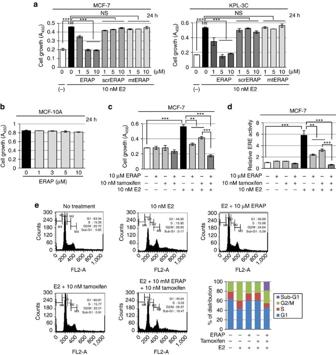Figure 5:ERAP suppresses growth of ERα-dependent breast cancer cell linesin vitro. (a,b) An MTT (3-(4,5-dimethylthiazol-2-yl)-2,5-diphenyltetrazolium bromide) assay was performed to evaluate the inhibitory effect of ERAP on E2-dependent growth of the BIG3-positive MCF-7 and KPL-3C (a), and the BIG3-negative mammary epithelial cell line MCF-10A (b). The data represent the mean±s.e.m. of three independent experiments (***P<0.001 in two-sided Student’st-test). (c,d) The combined inhibitory actions of ERAP and tamoxifen were evaluated using MTT assays (c) and luciferase assays (d). MCF-7 cells were treated for 24 h with E2±ERAP, tamoxifen, or a combination of ERAP and tamoxifen. The data of all panels represent the mean±s.e.m. of three independent experiments (**P<0.01, ***P<0.001 in two-sided Student’st-test). (e) Flow cytometric analyses were performed to evaluate the effect of ERAP treatment on the cell cycle. MCF-7 cells were treated for 24 h with E2±ERAP, tamoxifen, or a combination of ERAP and tamoxifen. Figure 5: ERAP suppresses growth of ERα-dependent breast cancer cell lines in vitro . ( a , b ) An MTT (3-(4,5-dimethylthiazol-2-yl)-2,5-diphenyltetrazolium bromide) assay was performed to evaluate the inhibitory effect of ERAP on E2-dependent growth of the BIG3-positive MCF-7 and KPL-3C ( a ), and the BIG3-negative mammary epithelial cell line MCF-10A ( b ). The data represent the mean±s.e.m. of three independent experiments (*** P <0.001 in two-sided Student’s t -test). ( c , d ) The combined inhibitory actions of ERAP and tamoxifen were evaluated using MTT assays ( c ) and luciferase assays ( d ). MCF-7 cells were treated for 24 h with E2±ERAP, tamoxifen, or a combination of ERAP and tamoxifen. The data of all panels represent the mean±s.e.m. of three independent experiments (** P <0.01, *** P <0.001 in two-sided Student’s t -test). ( e ) Flow cytometric analyses were performed to evaluate the effect of ERAP treatment on the cell cycle. MCF-7 cells were treated for 24 h with E2±ERAP, tamoxifen, or a combination of ERAP and tamoxifen. Full size image Furthermore, treatment with a combination of ERAP and tamoxifen significantly suppressed E2-induced cell growth ( Fig. 5c ) and ERα transcriptional activity ( Fig. 5d ) in MCF-7 cells as compared with ERAP or tamoxifen alone. Next, we examined the effects of ERAP on the cell cycle distribution of MCF-7 cells using flow cytometry. The population of cells in the G2/M phase increased after a 24 h E2 stimulation, whereas the population in the G1 phase increased after ERAP or tamoxifen treatment, suggesting that ERAP suppressed cell growth by inducing a G1 arrest, similar to tamoxifen [44] ( Fig. 5e ). Importantly, a remarkable increase in the apoptotic (sub-G1) cell population was observed after treatment with a combination of ERAP and tamoxifen (18.47%), although no phenotypic alterations or increases in the sub-G1 population were observed after treatment with ERAP, tamoxifen or E2 alone (0.29%, 0.91% or 0.17%, respectively; Fig. 5e ). Taken together, our data strongly suggest that ERAP enhanced the responsiveness of ERα-positive breast cancer cells to tamoxifen. Anti-tumour efficacy of ERAP in xenograft models To determine whether ERAP could affect the growth of ERα-positive breast cancer tumours in vivo , we developed KPL-3C ( Fig. 6a ) and MCF-7 ( Supplementary Fig. S6a ) orthotopic breast cancer xenografts in nude mice. Daily treatment with E2 alone induced time-dependent growth of KPL-3C and MCF-7 tumours, whereas treatment with 14 mg kg −1 ERAP caused significant inhibition of E2-induced tumour growth compared with mice treated with E2 alone or scrERAP in both tumour cell lines (14 mg kg −1 ; n =5; P <0.01 in two-sided Student’s t -test; Fig. 6a and Supplementary Fig. S6a ). No toxicity or significant body weight changes were observed in either xenograft throughout these experiments ( Supplementary Fig. S6b ). As expected, a significant reduction in mRNA levels was evident for TFF1 , CCND1 , and c-Myc in tumours treated with ERAP compared with those treated with scrERAP or vehicle only ( Fig. 6b and Supplementary Fig. S6c ). Furthermore, considerable suppression of Akt, p42/44 MAPK and ERα phosphorylation was observed in tumours treated with ERAP ( Fig. 6c and Supplementary Fig. S6d ). More importantly, the combined treatment of ERAP and tamoxifen additively inhibited the expression of ERα target genes ( Fig. 6b ) and the development of KPL-3C xenografts as compared with tamoxifen or ERAP alone ( Fig. 6a ). These results demonstrated that ERAP had in vivo anti-tumour activity and could enhance the anti-tumour effects of tamoxifen. 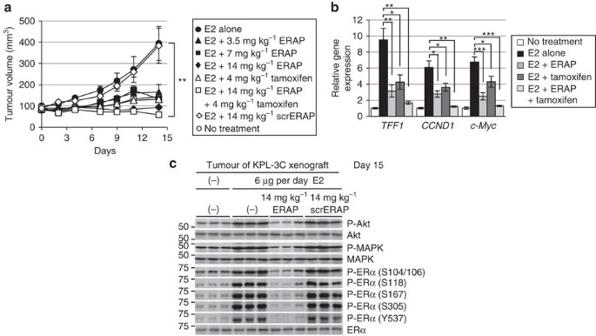Figure 6: ERAP inhibits tumour growth in xenograft models of human ERα-positive breast cancer. (a) ERAP inhibits tumour growth in a human breast cancer KPL-3C xenograft mouse model. The tumour volume represents the mean±s.e.m. of each group (n=5; **P<0.01 in two-sided Student’st-test). (b) Real-time PCR was performed to determine the combined inhibitory effects of ERAP and tamoxifen on the expression of ERα target genes. The data are expressed the fold increase over untreated cells at 0 h (set at 1.0) and represent the mean±s.e.m. of each group (n=5; *P<0.05, **P<0.01, ***P<0.001 in two-sided Student’st-test). (c) Immunoblot analyses were performed to evaluate the effects of ERAP on the phosphorylation levels of Akt, p42/44 MAPK and ERα proteins in tumours. Figure 6: ERAP inhibits tumour growth in xenograft models of human ERα-positive breast cancer. ( a ) ERAP inhibits tumour growth in a human breast cancer KPL-3C xenograft mouse model. The tumour volume represents the mean±s.e.m. of each group ( n =5; ** P <0.01 in two-sided Student’s t -test). ( b ) Real-time PCR was performed to determine the combined inhibitory effects of ERAP and tamoxifen on the expression of ERα target genes. The data are expressed the fold increase over untreated cells at 0 h (set at 1.0) and represent the mean±s.e.m. of each group ( n =5; * P <0.05, ** P <0.01, *** P <0.001 in two-sided Student’s t -test). ( c ) Immunoblot analyses were performed to evaluate the effects of ERAP on the phosphorylation levels of Akt, p42/44 MAPK and ERα proteins in tumours. Full size image ERAP suppresses growth of TAM-R tumours To confirm that ERAP had an anti-tumour effect against endocrine-resistant breast cancer, we first examined the effects of ERAP on the activation of the non-genomic signalling pathway, on the phosphorylation of ERα and on the non-canonical ERα transcriptional activation via AP-1, which is responsible for tamoxifen resistance [10] , [11] , [16] in TAM-R MCF-7 (ref. 45 ) and T47D (ref. 46 ) cells. The phosphorylation levels of Akt, p42/44 MAPK and ERα were enhanced in response to tamoxifen alone or a combination of tamoxifen and E2, whereas ERAP treatment clearly suppressed these responses in both cell types ( Fig. 7a,b and Supplementary Fig. S7a ). ERAP treatment also clearly suppressed the phosphorylation levels of Akt, p42/44 MAPK and ERα in response to a combination of E2 and IGF-2 in the presence of tamoxifen in TAM-R T47D cells ( Fig. 7b ). In addition, ERAP significantly inhibited E2-induced ERα transcriptional activity via AP-1, as well as ERE ( Supplementary Fig. S7b ), and the E2-induced expression of TFF1 , CCND1 and c- Myc genes ( Supplementary Fig. S7c,d ) in the presence of tamoxifen in TAM-R MCF-7 or TAM-R T47D cells. 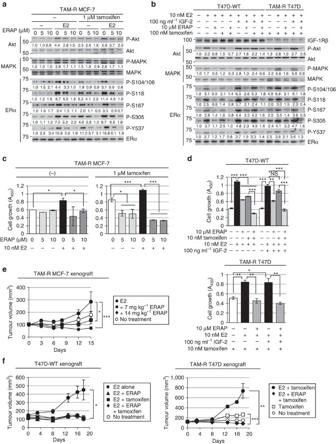Figure 7: ERAP suppresses growth of TAM-R tumours. (a,b) Immunoblot analyses were performed to evaluate the effects of ERAP on the phosphorylation levels of Akt, p42/44 MAPK and ERα proteins in TAM-R MCF-7 (a), and a parent T47D (T47D-WT) and TAM-R T47D (b) cells. (c) MTT (3-(4,5-dimethylthiazol-2-yl)-2,5-diphenyltetrazolium bromide) assays were performed to evaluate the inhibitory effect of ERAP on the growth of TAM-R MCF-7 cells. TAM-R MCF-7 cells were treated for 24 h with E2±ERAP in the presence or absence of 1 μM tamoxifen. The data represent the mean±s.e.m. of three independent experiments (*P<0.05, ***P<0.001 in two-sided Student’st-test). (d) Inhibitory effect of ERAP on the growth of T47D-WT (upper) and TAM-R T47D (lower) cells after 24 h of treatment with E2 alone or E2 and IGF-2 in the presence and the absence of 10 nM tamoxifen, respectively. The data of all panels represent the mean±s.e.m. of three independent experiments (*P<0.05, **P<0.01, ***P<0.001 in two-sided Student’st-test). (e) ERAP inhibits the tumour growth of TAM-R MCF-7 orthotropic breast cancer xenografts in nude mice. The tumour volume represents the mean±s.e.m. of each group (n=5) (*P<0.05, ***P<0.001 in two-sided Student’st-test). (f) ERAP inhibits the tumour growth of both T47D-WT (left) and TAM-R T47D (right) orthotropic breast cancer xenografts in nude mice. The tumour volume represents the mean±s.e.m. of each group (n=5; *P<0.05, **P<0.01, ***P<0.001 in two-sided Student’st-test). Figure 7: ERAP suppresses growth of TAM-R tumours. ( a , b ) Immunoblot analyses were performed to evaluate the effects of ERAP on the phosphorylation levels of Akt, p42/44 MAPK and ERα proteins in TAM-R MCF-7 ( a ), and a parent T47D (T47D-WT) and TAM-R T47D ( b ) cells. ( c ) MTT (3-(4,5-dimethylthiazol-2-yl)-2,5-diphenyltetrazolium bromide) assays were performed to evaluate the inhibitory effect of ERAP on the growth of TAM-R MCF-7 cells. TAM-R MCF-7 cells were treated for 24 h with E2±ERAP in the presence or absence of 1 μM tamoxifen. The data represent the mean±s.e.m. of three independent experiments (* P <0.05, *** P <0.001 in two-sided Student’s t -test). ( d ) Inhibitory effect of ERAP on the growth of T47D-WT (upper) and TAM-R T47D (lower) cells after 24 h of treatment with E2 alone or E2 and IGF-2 in the presence and the absence of 10 nM tamoxifen, respectively. The data of all panels represent the mean±s.e.m. of three independent experiments (* P <0.05, ** P <0.01, *** P <0.001 in two-sided Student’s t -test). ( e ) ERAP inhibits the tumour growth of TAM-R MCF-7 orthotropic breast cancer xenografts in nude mice. The tumour volume represents the mean±s.e.m. of each group ( n =5) (* P <0.05, *** P <0.001 in two-sided Student’s t -test). ( f ) ERAP inhibits the tumour growth of both T47D-WT (left) and TAM-R T47D (right) orthotropic breast cancer xenografts in nude mice. The tumour volume represents the mean±s.e.m. of each group ( n =5; * P <0.05, ** P <0.01, *** P <0.001 in two-sided Student’s t -test). Full size image Next, we tested the ability of ERAP to inhibit the E2-dependent growth of TAM-R cells and found that ERAP treatment significantly reduced the growth of TAM-R MCF-7 ( Fig. 7c ) and TAM-R T47D cells ( Fig. 7d ) in the presence of tamoxifen. Furthermore, we examined the inhibitory effects of ERAP on the E2-dependent tumour growth of TAM-R MCF-7 and T47D orthotropic breast cancer xenografts in nude mice. The results demonstrated that E2-induced growth of both TAM-R tumours was suppressed by treatment with 14 mg kg −1 ERAP ( n =4; P <0.001, Fig. 7e ; n =5; P <0.01 in two-sided Student’s t -test, Fig. 7f ). Furthermore, considerable suppression of Akt, p42/44 MAPK and ERα phosphorylation was observed in both TAM-R tumours treated with ERAP ( Supplementary Fig. S7e,f ). Collectively, these data suggested that ERAP acted as an effective therapeutic agent with respect to endocrine-resistant breast cancer. E2-dependent direct transactivation of BIG3 by ERα It was previously reported that BIG3 is upregulated after E2 treatment in MCF-7 cells [21] . Thus, we hypothesized that BIG3 may be a potential target gene of ERα and found that its expression was significantly upregulated in MCF-7 cells in a time-dependent manner after E2 stimulation ( Fig. 8a ). Interestingly, we also noted a significant reduction in BIG3 expression at both the transcriptional and protein levels in a dose-dependent manner after tamoxifen treatment ( Fig. 8b ). Accordingly, to obtain direct evidence for the upregulation of BIG3 expression by ERα, we measured ERα transcriptional activity. E2 stimulation resulted in robust luciferase activity only in cells transfected with the construct containing an intronic ERE from BIG3 ( Fig. 8c ), suggesting potential transactivation of BIG3 by ERα. Next, we examined the recruitment of ERα to an intronic ERE motif of the BIG3 gene by ChIP analysis ( Fig. 8d ). E2-dependent recruitment of ERα and the co-activator SRC-1 was observed associated with an ERE within intron 1 of the BIG3 gene in MCF-7 cells. In contrast, ERAP treatment enhanced recruitment of HDAC1 and NcoR to the ERα–PHB2 complex ( Fig. 8d ). In addition, ERAP treatment led to significant suppression of the E2-induced expression levels of BIG3 even after 3 h ( Fig. 8e ). These results demonstrated that BIG3 was directly transactivated by ERα via its intronic ERE following E2 treatment, which suggested that BIG3 acts through a positive feedback mechanism to enhance ERα activation in E2-dependent breast cancer cells. In other words, ERAP blocked this positive regulation of BIG3 , leading to the release of PHB2 from cytoplasmic BIG3 and the inhibition of ERα activity via multiple mechanisms. 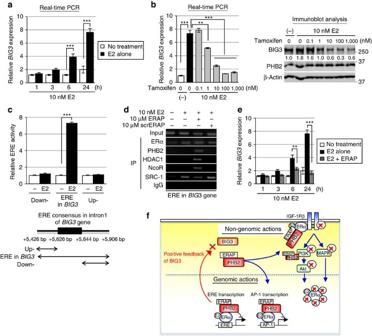Figure 8:Positive feedback regulation ofBIG3transactivation. (a) Upregulation ofBIG3expression was evaluated after E2 stimulation. These data are expressed the fold increase over untreated cells at 0 h (set at 1.0) and represent the mean±s.e.m. of three independent experiments (***P<0.001 in two-sided Student’st-test). (b) The effects of tamoxifen were evaluated onBIG3expression. For real-time PCR analyses (left), the data are expressed as the fold increase over untreated cells (set at 1.0). These data represent the mean±s.e.m. of three independent experiments (**P<0.01, ***P<0.001 in two-sided Student’st-test). For immunoblot analyses (right), β-actin served as a loading control. (c) Luciferase assays were performed to evaluate the transactivation ofBIG3using a luciferase reporter containing an ERE motif conserved within intron 1 of theBIG3gene (5′-TCCAGTTGCATTGACCTGA-3′; 5,626–5,644 bp from the transcriptional start site ofBIG3) or constructs containing the upstream and downstream regions lacking this ERE motif. The data represent the mean±s.e.m. of three independent experiments (**P<0.001 in two-sided Student’st-test). (d) ChIP assays show the transactivation ofBIG3through an intronic ERE. (e) The effect of ERAP onBIG3expression using real-time PCR is shown at the indicated time points. The data are expressed the fold increase over untreated cells at 0 h (set at 1.0) and represent the mean±s.e.m. of three independent experiments (**P<0.01, ***P<0.001 in two-sided Student’st-test). (f) ERAP treatment leads to multiple levels of inhibition targeted at E2-dependent ERα activation pathways. ERAP competitively binds to endogenous PHB2, thereby preventing its interactions with BIG3. Free PHB2 directly binds to both nuclear and membrane-associated ERα, resulting in the repression of E2-induced ERα activation through non-genomic pathways and its phosphorylation. Moreover, ERAP also attenuatesBIG3transcription, resulting in the downregulation of ERα target genes, includingBIG3. Figure 8: Positive feedback regulation of BIG3 transactivation. ( a ) Upregulation of BIG3 expression was evaluated after E2 stimulation. These data are expressed the fold increase over untreated cells at 0 h (set at 1.0) and represent the mean±s.e.m. of three independent experiments (*** P <0.001 in two-sided Student’s t -test). ( b ) The effects of tamoxifen were evaluated on BIG3 expression. For real-time PCR analyses (left), the data are expressed as the fold increase over untreated cells (set at 1.0). These data represent the mean±s.e.m. of three independent experiments (** P <0.01, *** P <0.001 in two-sided Student’s t -test). For immunoblot analyses (right), β-actin served as a loading control. ( c ) Luciferase assays were performed to evaluate the transactivation of BIG3 using a luciferase reporter containing an ERE motif conserved within intron 1 of the BIG3 gene (5′-TCCAGTTGCATTGACCTGA-3′; 5,626–5,644 bp from the transcriptional start site of BIG3 ) or constructs containing the upstream and downstream regions lacking this ERE motif. The data represent the mean±s.e.m. of three independent experiments (** P <0.001 in two-sided Student’s t -test). ( d ) ChIP assays show the transactivation of BIG3 through an intronic ERE. ( e ) The effect of ERAP on BIG3 expression using real-time PCR is shown at the indicated time points. The data are expressed the fold increase over untreated cells at 0 h (set at 1.0) and represent the mean±s.e.m. of three independent experiments (** P <0.01, *** P <0.001 in two-sided Student’s t -test). ( f ) ERAP treatment leads to multiple levels of inhibition targeted at E2-dependent ERα activation pathways. ERAP competitively binds to endogenous PHB2, thereby preventing its interactions with BIG3. Free PHB2 directly binds to both nuclear and membrane-associated ERα, resulting in the repression of E2-induced ERα activation through non-genomic pathways and its phosphorylation. Moreover, ERAP also attenuates BIG3 transcription, resulting in the downregulation of ERα target genes, including BIG3 . Full size image In this study, we developed a dominant-negative peptide, ERAP, based on the residues Q165, D169 and Q173 in BIG3, which were essential for its heterodimerization with PHB2 to suppress the growth of ERα-positive breast cancer cells, especially endocrine-resistant breast cancer cells. ERAP competitively bound endogenous PHB2, thereby preventing its interaction with BIG3 and releasing PHB2 to directly bind to both nuclear- and membrane-associated ERα. Intrinsic PHB2 binding to ERα led to the repression of a number of E2-induced activation events, which resulted in complete suppression of E2-dependent ERα-positive breast cancer cell growth in vitro and in vivo ( Fig. 8f ). These findings suggest that PHB2 has an important role in the modulation of multiple aspects of the E2/ERα-signalling network, although PHB2 has been reported to be the only transcriptional repressor for ERα. However, to date, it remains unclear how the endogenous tumour suppressor PHB2 is inactivated in cancer cells, despite abundant expression and the lack of genomic mutations or methylations in breast cancer clinical specimens or cell lines [47] . Our data suggest a potential solution to this unanswered problem; namely, our results suggest that BIG3 may sequester PHB2 in cancer cells, thereby causing an apparent ‘loss-of-function’ of PHB2 protein. These findings mark the first step toward uncovering a new E2/ERα signalling network in breast cancer and shed light on novel therapeutic strategies using PHB2 protein functions for E2/ERα-positive breast cancer. The most important finding of this study was that ERAP might potentially act as an effective inhibitor of TAM-R breast cancer cells. Current endocrine therapies for breast cancer are based mainly on targeting the ERα-signalling pathway, and tamoxifen is the most frequently prescribed drug for the treatment of all stages of breast cancer [12] , [13] . However, tamoxifen resistance is a major clinical problem and a leading cause of treatment failure and mortality [14] , [15] . Compelling evidence suggests that multiply phosphorylated ERα and non-canonical ERα activation via AP-1 are linked to tamoxifen or aromatase inhibitor resistance in breast cancer cells [10] , [11] , [16] . In addition, the activation of the IGF-1Rβ/AKT–ERK1/2–MAPK network is also linked to tamoxifen resistance in breast cancers [10] , [11] , [16] , even though the abundance of membrane-bound and cytoplasmic ERα is low in primary breast cancers [34] . Our study demonstrated that ERAP treatment completely inhibited ERα–IGF-1Rβ and/or ERα–PI3K interactions, ERα phosphorylation at multiple sites and ERα transcriptional activation via AP-1 in the presence of E2 in ERα-positive breast cancer cells. Indeed, ERAP had significant anti-tumour effects against TAM-R breast cancer cells. More importantly, we revealed that the combination of tamoxifen and ERAP induced rapid apoptosis and exhibited more potent anti-tumour activity in vivo and in vitro as compared with either treatment alone, indicating enhanced tamoxifen responsiveness. This combined effect is thought to be due to the distinct mechanisms of action of each drug, suggesting that releasing intrinsic PHB2 could suppress multifactorial mechanisms of endocrine resistance. Current endocrine therapies, such as tamoxifen, pinpoint specific signalling pathways or molecules in the ERα-signalling network. In contrast, ERAP was shown to modulate multiple aspects of the E2/ERα-signalling network via the tumour suppressive ability of endogenous PHB2, which was expressed abundantly in cancer cells, leading to the complete suppression of E2-dependent breast cancer cell growth. Moreover, although BIG3 is transactivated directly by ERα in a positive feedback loop, ERAP was shown to downregulate BIG3 transcription, which reduced BIG3 protein levels in the cytoplasm of cancer cells and enabled endogenous PHB2 to suppress the extensive ERα signalling network. Moreover, as BIG3 is specifically upregulated in breast cancer but is hardly detectable in normal human tissues, agents such as ERAP, which are designed to specifically disrupt BIG3 binding, may demonstrate excellent therapeutic indices with minimal off-target effects. Intracellular protein–protein interactions have been difficult to target with small molecules or synthetic peptide inhibitors, regardless of their ability to regulate many signalling networks. However, it has been reported that the Nutlins, selective small molecule antagonists of the MDM2–p53 interaction, possess in vitro and in vivo anti-tumour activity via the reactivation of p53 tumour suppressive activity [48] . In fact, as the inhibitory effect of ERAP was maintained for only 24 h ( Supplementary Fig. S5b ), it will be necessary to improve upon its pharmacologic properties using chemical synthetic approaches, such as hydrocarbon stapling methods [49] , [50] , or to screen selective small molecule antagonists targeting the BIG3–PHB2 interaction. In conclusion, targeting the BIG3–PHB2 interaction represents a potential new treatment avenue for ERα-positive breast cancer patients. This new approach could be an important supplement therapy and may provide mechanistic insight into the molecular basis of ERα-signalling networks in breast carcinogenesis. Thus, combining endocrine treatment with these new targeted therapies is a promising approach for improving the current treatment strategies and overcoming endocrine resistance, and should be investigated in future preclinical and clinical studies. ERα antibody The anti-ERα (clone AER314) antibody was purchased from Thermo Fisher Scientific (Fremont, CA). This antibody specifically recognizes undigested ERα and is equivalent to an anti-ERα antibody (SP-1) [34] , which is widely used for immunohistochemical analysis ( Supplementary Fig. S8 ). Immunoblot analyses Cells were lysed with lysis buffer (50 mM Tris-HCl, pH 8.0; 150 mM NaCl, 0.1% NP-40, 0.5% CHAPS) containing 0.1% protease inhibitor cocktail III (Calbiochem, San Diego, CA). The lysates were electrophoretically separated, blotted onto a nitrocellulose membrane and blocked with 4% BlockAce solution (Dainippon Pharmaceutical, Osaka, Japan) for 1 h. The blots were then incubated with antibodies against the following proteins: BIG3 (ref. 21 ) (1:200); PHB2 (1:500), NcoR (1:500) and ERα (phospho Y537; 1:500; Abcam, Cambridge, UK); SRC-1 (128E7; 1:500), Shc (1:500), α/β-tubulin (1:1,000), Akt (1:1,000), phospho-Akt (S473; 587F11; 1:1,000), p44/42 MAPK (1:500), phospho-p44/42 MAPK (T202/Y204; 1:500) and phospho-ERα (S104/S106; 1:500; Cell Signaling Technology, Danvers, MA); HDAC1 (H-11; 1:500), IGF-1Rβ (1:500), PI3-kinase p85α (U13; 1:500), phospho-ERα (S118; 1:500), phospho-ERα (S167; 1:500) and laminin B1 (1:100; Santa Cruz Biotechnology, Santa Cruz, CA); phospho-ERα (S305; 1:500; Millipore, Billerica, MA); phosphotyrosine (1:500; Zymed, San Francisco, CA); β-actin (AC-15; 1:5,000) and FLAG-tag M2 (1:5,000; Sigma, St Louis, MO); and HA-tag (1:3,000; Roche, Mannheim, Germany). After incubation with an horseradish peroxidase-conjugated secondary antibody (Santa Cruz Biotechnology, dilution 1:5,000) or monoclonal anti-rabbit immunoglobulins-peroxidase antibody (RG-16, Sigma, dilition 1:5,000) for 1 h, the blots were developed with an enhanced chemiluminescence system (GE Healthcare, Buckinghamshire, UK) and were scanned using an Image Reader LAS-3000 mini (Fujifilm, Tokyo, Japan). All experiments were performed more than three times in triplicate. Finally, the phosphorylation levels of IGF-1Rβ, Shc, PI3K, Akt, p42/44 MAPK and ERα were assessed through densitometric analysis of immunoblot results using an Image Reader LAS-3000 mini [51] . Full-length images of immunoblots are shown in Supplementary Fig. S9 . Immunoprecipitation The cells were lysed with 0.1% NP-40 lysis buffer as described above. The cell lysates were precleared with normal IgG and rec-Protein G Sepharose 4B (Zymed) at 4 °C for 3 h. Then, the supernatants were incubated with antibodies against BIG3 (5 μg), PHB2 (5 μg) and ERα (5 μg) at 4 °C for 12 h. Next, the antigen–antibody complexes were precipitated with rec-Protein G Sepharose 4B at 4 °C for 1 h. Immunoprecipitated protein complexes were washed three times with lysis buffer and separated using SDS–PAGE. Immunoblot analyses were performed as described above. Identification of the PHB2-binding regions in BIG3 protein To determine the PHB2-binding region in BIG3, we cloned five different constructs corresponding to partial BIG3 sequences (BIG3 1–434 , BIG3 435–2,177 , BIG3 1,468–2,177 , BIG3 1–100 and BIG3 1–250 ) into an amino-terminal FLAG-tagged pCAGGS vector. COS-7 cells were individually cotransfected with a BIG3 vector and HA-PHB2 using the FuGENE6 transfection reagent (Roche). At 48 h after transfection, the cells were lysed with 0.1% NP-40 lysis buffer. The lysates were precleared for 3 h at 4 °C and then incubated with anti-FLAG M2 agarose (Sigma) for 12 h at 4 °C. Next, the immunoprecipitated proteins or intact cell lysates were electrophoresed and blotted onto nitrocellulose. Finally, the blots were incubated with antibodies against FLAG M2 or HA-tag. Interaction site and structure prediction BIG3 and PHB2 interaction sites were predicted using PSIVER. PSIVER is a computational method to predict residues that bind to other proteins using only sequence features (position-specific scoring matrix and predicted accessibility). The method uses the Naive Bayes classifier with kernel density estimation and was shown to outperform existing servers available on the Internet. The default threshold of 0.390 was used in this study. Structure prediction was performed using FUGUE [52] and PSIPRED [53] . A model of the putative PHB2-binding helix of BIG3 (residues 157–174) was built using MODELLER [54] based on the TIP120 protein [55] as a template. BIG3–PHB2 interaction inhibition by ERAP The 13 amino acid peptides derived from the PHB2-binding domain of BIG3 (codons 165–177) were covalently linked at the NH 2 terminus to a membrane transducing 11 polyarginine sequence (11R) to construct the ERAP peptide. Negative control peptides, scrERAP and mtERAP, were also synthesized. To examine the effects of ERAP on inhibition of BIG3–PHB2 complex formation, MCF-7 cells were treated with 10 nM E2±10 μM ERAP. BIG3–PHB2 interactions were assessed using co-immunoprecipitation followed by immunoblotting, as described above. Nuclear/cytoplasmic fractionation MCF-7 cells were treated as described above, and nuclear and cytoplasmic/plasma membrane fractions were prepared using the NE-PER nuclear and cytoplasmic extraction reagent (Thermo Fisher Scientific) according to the manufacturer’s instructions. α/β-Tubulin and laminin B were used as loading controls for the cytoplasmic and nuclear fractions, respectively. Cell proliferation assay Cell proliferation assays were performed using the Cell Counting Kit-8 (Dojindo, Kumamoto, Japan). The cells were plated in 48-well plates at 2 × 10 4 cells per well and maintained at 37 °C. At the indicated time points, a 1:10 dilution of the Cell Counting Kit-8 solution was added (into three replicate wells) and incubated for 1 h. Then, the absorbance at 450 nm was measured to calculate the number of vital cells per well. The data represent the mean±s.e.m. of three independent experiments. In vivo tumour growth inhibition Each suspension (1 × 10 7 cells per mouse) of KPL-3C cells, MCF-7 cells, T47D cells, TAM-R MCF-7 cells or TAM-R T47D cells was mixed with an equal volume of Matrigel (BD, Franklin Lakes, NJ) and injected (200 μl total) into the mammary fat pads of 6-week-old female BALB/c nude mice (Charles River Laboratories, Tokyo, Japan). The mice were housed in a pathogen-free isolation facility with a 12-h light/dark cycle, and were fed rodent chow and water ad libitum . The tumours developed over a period of 1 week, reaching sizes of ~100 mm 3 (calculated as 1/2 × (width × length 2 )). For KPL-3C orthotropic xenograft experiments, the mice were randomized into eight treatment groups (five animals per group): (1) no treatment; (2) 6 μg per day E2; (3–5) E2+3.5, 7 or 14 mg kg −1 per day ERAP; (6) E2+14 mg kg −1 per day scrERAP; (7) E2+4 mg kg −1 per day tamoxifen; and (8) E2+4 mg kg −1 per day tamoxifen+14 mg kg −1 per day ERAP. For the MCF-7 orthotopic xenograft, the mice were randomized into three treatment groups: (1) 6 μg per day E2; (2) E2+14 mg kg −1 per day ERAP; and (3) E2+14 mg kg −1 per day scrERAP. For the T47D orthotopic xenograft, the mice were randomized into five treatment groups: (1) no treatment; (2) 6 μg per day E2; (3) E2+14 mg kg −1 per day ERAP; (4) E2+3.7 μg kg −1 per day tamoxifen; and (5) E2+ERAP+tamoxifen. For TAM-R MCF-7 orthotropic xenograft, the mice were randomized into four treatment groups: (1) no treatment; (2) 37 μg kg −1 per day tamoxifen; (2) 6 μg per day E2+tamoxifen; and (3, 4) E2+tamoxifen+7 or 14 mg kg −1 per day ERAP. For TAM-R T47D orthotopic xenografts, the mice were randomized into four treatment groups: (1) no treatment; (2) 3.7 μg kg −1 per day tamoxifen; (3) 6 μg per day E2+tamoxifen; and (4) E2+ tamoxifen+14 mg kg −1 per day ERAP. E2 was delivered via the application of a solution to the skin at the neck; the other treatments were delivered via intraperitoneal injection. Tumour volume was measured with calipers for 2 weeks, after which time the animals were killed, and the tumours were excised and frozen in liquid nitrogen. All experiments were performed in accordance with the guidelines of the animal facility at the University of Tokushima. For evaluations of the inhibitory effects of ERAP on tumour expression of ERα target genes using real-time PCR, the data are expressed as the fold increase in gene expression over the no treatment group (set at 1.0) and represent the mean±s.e.m. of each group (five mice). In addition, for evaluations of the effects of ERAP on the phosphorylation of Akt, p42/44 MAPK and ERα proteins in tumours, each tumour lysates (three to four mice per group) was immunoblotted. Statistical analyses A Student’s t -test was used to determine the significance of differences among the experimental groups. Values of P <0.05 were considered significant. The other methods are described in Supplementary Information . How to cite this article: Yoshimaru, T. et al. Targeting BIG3–PHB2 interaction to overcome tamoxifen resistance in breast cancer cells. Nat. Commun. 4:2443 doi: 10.1038/ncomms3443 (2013).